Temperature-dependent elastic anisotropy and mesoscale deformation in a nanostructured ferritic alloy Nanostructured ferritic alloys are a new class of ultrafine-grained oxide dispersion-strengthened steels that have promising properties for service in extreme environments in future nuclear reactors. This is due to the remarkable stability of their complex microstructures containing numerous Y-Ti-O nanoclusters within grains and along grain boundaries. Although nanoclusters account primarily for the exceptional resistance to irradiation damage and high-temperature creep, little is known about the mechanical roles of the polycrystalline grains that constitute the ferritic matrix. Here we report an in situ mesoscale characterization of anisotropic responses of ultrafine ferrite grains to stresses using state-of-the-art neutron diffraction. We show the experimental determination of single-crystal elastic constants for a 14YWT alloy, and reveal a strong temperature-dependent elastic anisotropy that leads to elastic softening and instability of the ferrite. We also demonstrate, from anisotropy-induced intergranular strains, that a deformation crossover exists from low-temperature lattice hardening to high-temperature lattice softening in response to extensive plastic deformation. For high-temperature applications, polycrystalline grains can be detrimental in structural materials, such as Ni-based superalloys, but they are beneficial for creep-resistant nanostructured ferritic alloys (NFAs) [1] , [2] , [3] . The ultrafine grains in NFAs remain unusually stable with little or no grain growth, coarsening or recrystallization up to 800–900 °C. Although nanoclusters (NCs) and precipitates that are embedded in the grains and along the grain boundaries [4] , [5] , together with solute segregation of W and Cr to the grain boundaries, are widely recognized to account for the excellent creep resistance [2] , [4] , [6] , [7] , [8] , the ultrafine ferrite grains are also essential in promoting the mechanical strength, for example, via Hall-Petch hardening [9] . Thus, it is important to understand how the ferrite grains deform in response to stresses, particularly, at elevated temperatures. When subjected to an applied load, each grain in a polycrystalline NFA behaves like a single crystal. It is known that a single crystal exhibits elastic and plastic anisotropy, as its elastic stiffness and plastic strength depend on the crystallographic orientation. The mechanical response of a NFA grain, within a polycrystalline NFA aggregate, is dependent on its single-crystal properties, the crystallographic orientation of its lattice and those of its neighbouring grains [10] . In particular, iron and its alloys are among the most anisotropic body-centred cubic metals, for instance, <111> is the stiffest orientation that is ~2.2 times as strong as the most compliant <100> orientation [11] . As such, in response to loading, differently oriented NFA grains will sustain distinctly different elastic strains and thus generate intergranular strains to maintain compatibility with its neighbouring grains [10] , [12] . Plastic deformation starts within grains whose orientation, relative to the loading axis, facilitates the easy activation of their dislocation slip systems when the critical resolved shear stress is reached; other oriented grains, which are plastically hard, will respond to the load elastically and sustain more loads leading to stress redistribution among the grains. In the case of uniaxial tensile loading, the plastically deformed grains accumulate a compressive intergranular strain, whereas the grains lying along the plastically hard orientations accommodate a tensile intergranular strain [10] , [13] . Thus, elastic anisotropy plays a predominant role in the early stage of plastic deformation, particularly for the orientation dependence of dislocation slip activity [14] , while the anisotropy-induced intergranular strains contain unique information about the dislocation activities and on the deformation processes [12] , [13] , [15] , [16] . As such, it is imperative to determine the elastic anisotropy and intergranular strains of NFAs to understand their grain-level anisotropic deformation behaviours. In this study, we have characterized in situ the mesoscale anisotropic responses of selected grains in a 14YWT NFA to uniaxial tensile loading at a broad range of temperatures, by state-of-the-art neutron diffraction at the Spallation Neutron Source (SNS), Oak Ridge National Laboratory. From the responses to elastic deformation, the single-crystal elastic constants of 14YWT were determined by considering the effect of preferred grain orientations (or texture), showing a strong temperature-dependent elastic anisotropy. From those in response to extensive plastic deformation that manifest anisotropy-induced intergranular strains, a deformation crossover was evident from a low-temperature intragranular dislocation slip mechanism to that mediated by grain boundary activities at elevated temperatures. Tensile deformation at elevated temperatures The material used in the present study was the ultrafine-grained 14YWT NFA with a nominal composition of Fe-14Cr-0.16W-0.4Ti-0.14Y-0.4O (at.%) (see alloy synthesis in Methods). Atom probe tomography and transmission electron microscopy characterizations showed that the 14YWT NFA has a grain size of 200–400 nm and contains a high number density of Y-Ti-O NCs (1-2 nm in diameter) inhomogeneously distributed in the grains and along the grain boundaries [4] , [17] . As the alloy was made by hot-extrusion of mechanically alloyed powders, the 14YWT NFA tensile specimen exhibits a strong <110> fibre texture, as seen from the neutron diffraction patterns and also consistent with the texture characterization in earlier works [18] . In situ neutron diffraction characterization of the 14YWT NFA under uniaxial tensile loading at room temperature (RT), 400, 600, 750 and 800 °C, respectively, was performed on VULCAN [19] , the Engineering Materials Diffractometer at the SNS (see Methods, Supplementary Figs 1–4 and Supplementary Note 1 for more details of the experimental setup). The observed true stress–true strain curve at each temperature is shown in Fig. 1a , and selected diffraction patterns collected during tensile loading at RT are presented in Fig. 1b,c . The neutron scattering geometry (see Supplementary Fig. 1 ) allows for simultaneous measurements of two scattering vectors Q 1 and Q 2 , which are parallel and perpendicular to the tensile axis, respectively. Diffraction from the crystal lattice of grains whose plane normal (that is, < hkl >) is parallel to Q 1 or Q 2 and satisfies Bragg’s law will be detected, and the lattice spacing ( d hkl ) can thus be measured from the diffraction peak corresponding to the ( hkl ) reflection. If treating the crystal lattice as a natural ‘atomic plane strain gauge’, lattice strains are determined from the shifts of lattice spacing due to an applied load, that is, where is the stress-free reference lattice spacing. Accordingly, two lattice strain components, one parallel to the tensile axis (that is, the loading direction, LD) and the other perpendicular to the tensile axis (that is, the transverse direction, TD), are measured simultaneously under tensile loading. As the macroscopic stress is uniaxial, only one stress component value is different from zero ( σ 3 ≠ 0, LD → 3, TD → 1 where 1–3 refer to the three orthogonal axes). The two components of the grain-orientation-dependent strains recorded by our experimental setup are designated as ε 3 ( hkl ) for the LD and ε 1 ( hkl ) for the TD. The generic hkl indices denote not only a measurement direction in the crystal space, but also refer to specific families of grain orientation. The family of grains whose plane normal < hkl > lies along the LD or the TD is designated as < hkl >//LD or < hkl >//TD, respectively. 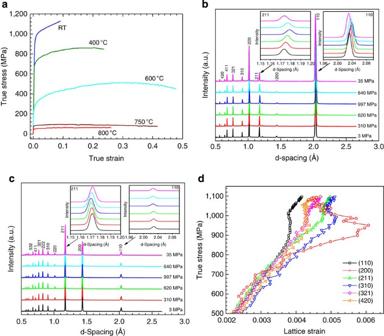Figure 1: Strain measurements byin situneutron diffraction. (a) True stress–true strain curves for tensile loading of the 14YWT NFA at RT, 400, 600, 750 and 800 °C, respectively. (b,c) Selected neutron diffraction patterns collected with respect to the loading and transverse directions during tensile loading of an NFA at RT for a loading-unloading cycle (from bottom to top). (d) True stress–lattice strain curves for six <hkl>//LD families of grains obtained during tensile loading at RT. Figure 1d shows the variation of true stress with the lattice strain for six < hkl >//LD families of grains obtained during tensile loading at RT. Thus, neutron diffraction serves as a grain selector and can provide unique insights into the grain-scale deformation mechanisms. Figure 1: Strain measurements by in situ neutron diffraction. ( a ) True stress–true strain curves for tensile loading of the 14YWT NFA at RT, 400, 600, 750 and 800 °C, respectively. ( b , c ) Selected neutron diffraction patterns collected with respect to the loading and transverse directions during tensile loading of an NFA at RT for a loading-unloading cycle (from bottom to top). ( d ) True stress–lattice strain curves for six < hkl >//LD families of grains obtained during tensile loading at RT. Full size image Crystallographic texture Beside lattice-spacing shifts, diffraction peaks can be used to assess the preferred orientation of grains (or texture). A virtual population of randomly oriented single crystals, generated by the quasi-Monte Carlo method, facilitates the realistic calculation of weighting factors for different powder diffraction peaks detected by each of the two instrument detector banks at VULCAN, as well as the correlation between the peaks recorded in different banks. The integrated intensities of a few independent diffraction peaks, after normalization to respective intensities obtained from a reference sample with random textures, are chosen to generate inverse pole figures (IPFs) with respect to the LD and TD. For a BCC structure, nine crystallographic directions define a network for texture index estimations, and the fundamental triangle is partitioned in eight triangular cells (see Supplementary Fig. 5 ). The texture index inside each cell is defined using a barycentric interpolation method (see more details in Supplementary Note 2 ). As the initial texture of the NFA specimens is expected to have the axial symmetry due to hot extrusion, and the tensile deformation preserves the same symmetry, the IPFs allow for a complete texture description and can be efficiently used for averaging procedures in the analysis of stresses and strains. Two IPF maps with respect to the LD and TD are depicted in Fig. 2a,b , respectively, showing clearly the presence of a strong <011> fibre texture in the NFA specimens before tensile loading (see more IPFs in Supplementary Figs 6 and 7 ). Under tensile loading, the <011>//LD fibre texture underwent a moderate strengthening. 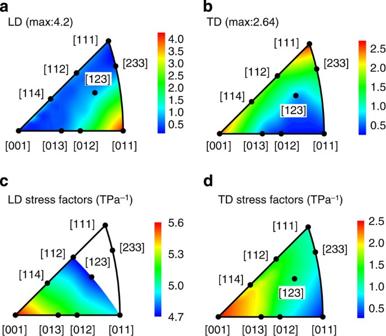Figure 2: Texture characterization and stress-factor determination. Inverse pole figures with respect to (a) LD and (b) TD for the NFA before tensile loading, showing the strong presence of a <110//LD> fibre texture. Stress-factor inverse pole figures with respect to (c) LD and (d) TD for the NFA tensile loaded at 400 °C. Figure 2: Texture characterization and stress-factor determination. Inverse pole figures with respect to ( a ) LD and ( b ) TD for the NFA before tensile loading, showing the strong presence of a <110//LD> fibre texture. Stress-factor inverse pole figures with respect to ( c ) LD and ( d ) TD for the NFA tensile loaded at 400 °C. Full size image Stress factors and single-crystal elastic constants To illustrate the elastic anisotropy and intergranular strain accumulations in the NFA, the evolution of the lattice strains ε 3 ( hkl ) of several families of grains (< hkl >//LD) under RT tensile loading has been shown in Fig. 1d . In the elastic regime, the lattice strain is linear as a function of the applied stress ( σ 3 ), where the slope represents the elastic stiffness at the grain level and manifests the effect of cubic elastic anisotropy. Upon plastic deformation, the lattice strain begins to deviate from the elastic linearity and this effect is irreversible. The difference between the current value of lattice strain and the value extrapolated from the elastic response (that is, the reversible part of the lattice strain) is termed as intergranular strain as mentioned earlier, or Type II strain (ref. 11 ) and is conceptually equivalent with the residual strain recorded after unloading elastically from the current level of stress. In the following sections, the focus is placed on analyzing the linear regime of the lattice strain evolution, in order to determine the single-crystal elastic constants that give rise to the elastic anisotropy at different temperatures. In diffraction stress analysis for polycrystalline aggregates, there are two ways of approaching the strain response at the grain level. The first considers the proportionality between the grain-level average normal strain components (measured by diffraction along certain single crystal directions) and the macroscopic stress components applied at the specimen level. The proportionality factors are defined as ‘stress factors’. They can be calculated starting from single-crystal elastic constants by taking into account the crystallographic texture and orientation stereology (that is, grain shape and packing) using various averaging techniques [20] , [21] , [22] , [23] , [24] . This approach was also consistently used to retrieve the single-crystal elastic constants from polycrystalline diffraction data, especially when the texture influence is absent or weak. The second approach has been developed as a tool for residual stress determination in deformed specimens after the external load is released. The macroscopic stress components are not known in this case; it is thus necessary to define a mesoscopic average stress field depending on the grain orientations, known as the stress orientation distribution function [25] , [26] , [27] , [28] . In this case, the proportionality factors between the strain and stress components are fully determined by the single-crystal elastic constants, although additional restrictive conditions or grain interaction models are often needed to obtain physically consistent solutions for the stress field. In the present work, as the NFA specimens exhibit a strong <110> fibre texture as demonstrated in the preceding section, the second approach has been applied to retrieve the single-crystal elastic constants from the in situ neutron diffraction data. In this approach, the orientation-dependent stress acting at the grain level is a free parameter, but, to reduce the number of parameters, the average local stress is considered to be uniaxial and parallel to the applied stress [29] . The FEM simulation results reported by ref. 10 seem to support this assumption. As the analysis of lattice strains was performed in the elastic region only, the experimentally determined stress factors were used as inputs in the model, while elasticity equations for single-crystals with cubic symmetry were applied for uniaxial straining [30] . In the elastic regime, the longitudinal lattice strain component, ε 3 ( hkl ), is related to the applied stress through the stress factor F 33 ( hkl ), The transverse lattice strain, ε 1 ( h ′ k ′ l ′), can be represented as a sum of transversally isotropic fibres with the < h i k i l i > orientation along the LD, where w i is the volume fraction of the i th fibre, f i ( h ′ k ′ l ′) the probability of grains belonging to the i th fiber that has the < h ′ k ′ l ′> direction along the TD, F 13 ( h ′ k ′ l ′, h i k i l i ) the stress factor for grains with < h ′ k ′ l ′> along the TD and < h i k i l i > along the LD, and > the average transverse stress factor. The average transverse stress factor, , or the longitudinal stress factor, F 33 ( hkl ), can be determined from the slopes of the lattice strain [ ε 1 ( h ′ k ′ l ′) or ε 3 ( hkl )] versus true stress curves recorded during loading or unloading in the elastic regime of deformation. Because of the strong initial <110> texture (that is, ~50% of the grains are oriented as <011>//LD), only six longitudinal stress factors could be determined in the present work, and this number amounts to eight for the transverse stress factors. The hkl stress factor distribution can be represented as an IPF map. For instance, the stress factor IPFs collected at 400 °C are shown in Fig. 2c,d for LD and TD, respectively (see Supplementary Figs 8–10 and Supplementary Note 3 for other temperatures). The experimental values of stress factors were obtained from averaging the measured slopes recorded during a few (2–4) loading/unloading cycles, as a systematic drift with the degree of plastic deformation was not discernible (that is, slow texture development during loading). Stress factors can be calculated based on the single-crystal elasticity and by considering the adjustable stress concentration factors that link the local stress field to the applied stress. As such, equations (1) and (2) can be written as where p i are the average stress concentration factors attached to different texture fibres and In the above equations, n i and m i are the hkl and h ′ k ′ l ′ direction cosines in the cubic lattice cell, S ij and c ij the coefficients of compliance and stiffness for the single crystal, and A the anisotropy parameter. The basic fibres include <110>, <200>, <211>, <310>, <222>, <321>, <411>, <420> and <332> along the LD, which are given in Supplementary Note 2 and represented in Supplementary Fig. 5 . As the main fibre component contained almost 50% of the grains aligned with the <011> generic direction along the LD, the p i values were treated differently for <011> and the rest of the components. The p i corresponding to minor components (<001>, <013>, <012>, <112> and <123>) were correlated through a rational function of F ( n ) and the weighted average over all the p i values was constrained to 1 (that is, the average stress is identical to the applied true stress). The values of single-crystal elastic constants were adjusted to minimize the squared difference between the experimental stress factors values and the calculated ones. The IPFs were used to determine the volume fractions w i and the correlation factors f i ( m j ). Although the influence of texture is generally challenging to quantify, the <011>//LD fibre texture, in this NFA, indeed facilitated the observation of the distinct difference in the transverse stress factors between the <011> and <112> directions, as illustrated in Fig. 3 . Following equation (4), if the tensile load is applied along the <110> direction, D(n,m) varies from ½ to 0 and the corresponding transverse compliances change from positive to negative (see Fig. 3a ). For ferritic steels, this peculiarity was recognized by ref. 31 . Because of the strong <011>//LD fibre texture, in our case, the transverse stress factor for the <110> direction can effectively go positive for large elastic anisotropy ( Fig. 3b ). The single-crystal cubic elastic constants, c 11 , c 12 and c 44 , have been deduced from the single-crystal compliances ( S ij ) by matching the experimental and calculated stress factors; these values, together with the shear stiffness [ c ′=( c 11 − c 12 )/2] and the elastic anisotropy parameter ( A ), are listed as a function of temperature in Table 1 and also shown in Fig. 4 . Our estimation of relative errors of S 11 , S 12 and S 44 amounts to 2% or less for RT, 400 and 600 °C, but increases to 5% or more for 750 and 800 °C. A strong temperature-dependent c ′ and A are evident as expected from those of pure Fe, which will be discussed in greater detail below. 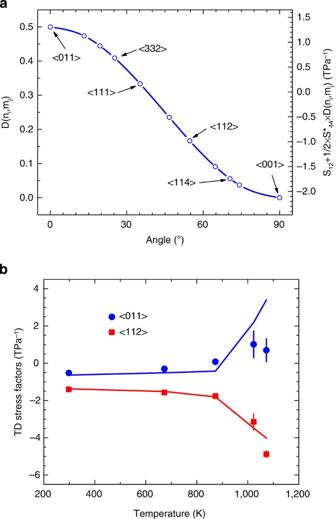Figure 3: Elastic anisotropy of transverse stress factors. (a) Geometric factor D in equation (4) (left axis) and the transverse anisotropy at RT (right axis) as a function of angle towards the <011> direction, and (b) Temperature dependence of transverse stress factor for the <011> and <112> directions. Symbols and lines inbdenote experimental and calculated values, respectively. Figure 3: Elastic anisotropy of transverse stress factors. ( a ) Geometric factor D in equation (4) (left axis) and the transverse anisotropy at RT (right axis) as a function of angle towards the <011> direction, and ( b ) Temperature dependence of transverse stress factor for the <011> and <112> directions. Symbols and lines in b denote experimental and calculated values, respectively. Full size image Table 1 Temperature-dependent mechanical properties. 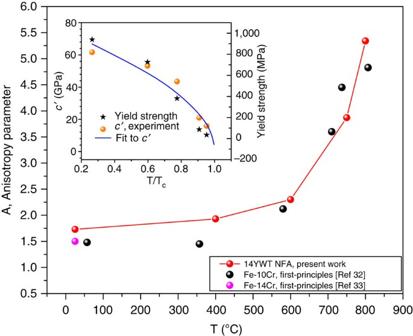Figure 4: Temperature-dependent anisotropy parameter. Comparison of the temperature-dependent anisotropy parameters (A) experimentally determined in the present work with those obtained from first-principles calculations by refs32,33. The inset showsc′ and the 0.2% yield stress as a function of temperature. Full size table Figure 4: Temperature-dependent anisotropy parameter. Comparison of the temperature-dependent anisotropy parameters ( A ) experimentally determined in the present work with those obtained from first-principles calculations by refs 32 , 33 . The inset shows c ′ and the 0.2% yield stress as a function of temperature. Full size image Intergranular strains and mesoscale deformation As indicated in Fig. 1d , the <110>//LD grains are the first to yield and then take on compressive intergranular strains on plastic deformation at RT. This is also the case for other higher temperatures. The intergranular strain accumulation in the <110>//LD grains thus contains mesoscale information characteristic of the plastic deformation. In what follows, we show how the <110> intergranular strain accumulates as plastic deformation proceeds at various temperatures, which provide insights into the deformation mechanisms. The applied true stresses as a function of lattice strain of the <110>//LD grains obtained at RT, 400, 600, 750 and 800 °C, respectively, are shown in Fig. 5 . Intergranular strains (Δ ε II ) accumulated in the <110>//LD grains (see the upper left inset of Fig. 5 ) are calculated by subtracting the current lattice strain ( ε ) from the projected linear elastic strain corresponding to the current applied stress ( σ ), that is, where is the slope of the σ versus ε curve in the elastic regime at the temperature T . Normalized intergranular strain ( ) as a function of normalized true stress ( ) for each of the five temperatures has been plotted in the lower right inset of Fig. 5 , where is defined as the yield stress necessary for the <110>//LD grains to induce a plastic strain of 50 × 10 −6 and is the corresponding lattice strain. At low temperatures (RT and 400 °C), the <110> intergranular strain was accumulated gradually and became saturated at a value of when the applied true stress increased continuously over ; this clearly depicts the initial yielding of the <110>//LD grains (fixed lattice strain and taking no more loads) followed by strain hardening (increased lattice strain and taking on loads elastically). At the intermediate temperature (that is, 600 °C), the intergranular strain accumulation appears to be similar to what underwent at low temperatures and also turned to be saturated but at a higher value of ; however, in sharp contrast, the intergranular strain saturation continued with a decrease in the applied true stress from a value of . This behaviour indicates a mechanism of initial yielding followed by strain softening due to extensive plastic deformation. At high temperatures (750 °C and 800 °C), intergranular strains were accumulated immediately after the onset of yielding but, strikingly, with the decrease in the applied true stress, indicative of strain softening. 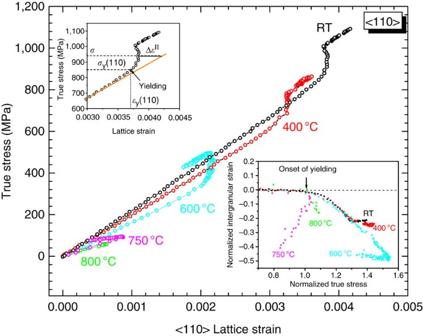Figure 5: Evolution of intergranular strains. Applied true stress as a function of the <110> lattice strain at various temperatures. The inset at the upper-left corner shows the onset of yielding (corresponding to a plastic strain of 50 με), and the definition of type II intergranular strain (ΔεII). The inset at the lower-right corner represents normalized <110> intergranular strain as a function of normalized true stress for different temperatures during plastic deformation. Figure 5: Evolution of intergranular strains. Applied true stress as a function of the <110> lattice strain at various temperatures. The inset at the upper-left corner shows the onset of yielding (corresponding to a plastic strain of 50 μ ε ), and the definition of type II intergranular strain (Δ ε II ). The inset at the lower-right corner represents normalized <110> intergranular strain as a function of normalized true stress for different temperatures during plastic deformation. Full size image The experimentally determined anisotropy parameter ( A ) is shown in Fig. 4 as a function of temperature ( T ), which agrees remarkably well with the predictions obtained from first-principles calculations by refs 32 , 33 . This result validates the above-mentioned method that was developed to extract elastic constants from textured polycrystalline materials. The marked increase in A at elevated temperatures is attributed to a sudden drop of the shear stiffness constant ( c ′) as T approaches a critical value (T c ); this has been depicted in the inset of Fig. 4 , together with a best fit to the experimental data by the function: . T c is determined to be 1,127 K (854 °C) for the NFA, in comparison with that of 1,185 K (912 °C) for pure Fe with (ref. 34 ). For pure Fe, T c is the bcc-fcc or α - γ transition temperature as proved by ref. 34 . The displacive α - γ transition has been found to be associated with the development of the (110) soft transverse acoustic phonon mode, corresponding to shear deformation of the BCC unit cell along the phase transformation pathway [34] , [35] , [36] , [37] . For the 14YWT NFA, however, the α - γ transition and the presence of T c are unexpected. Nevertheless, this transition was experimentally observed in the in situ neutron diffraction studies of a 14YWT NFA, which showed a face-centred cubic γ -phase occurring at ~910 °C and then disappearing at ~810 °C when cooling from 1,300 °C to RT (see Supplementary Fig. 11 ). This transition is likely when considering the Fe-Cr binary phase diagram, which exhibits an ( α + γ ) two-phase region between 11.2 wt.% Cr and 13.4 wt.% Cr ranging from ~846 °C up to 1,200 °C. Additions of other alloying elements (for example, Y and Ti, and so on.) appear to widen the ( α + γ ) region; this makes 14YWT lying, most likely, in the vicinity of the α /( α + γ ) boundary, as indicated by the observed small volume fraction (that is, <1.5%) of the transformed γ from neutron diffraction. Thus, the α - γ transition in 14YWT appears to be marginal. However, no matter how small the transformed- γ amount is, the phase transition, if present, kinetically requires the whole α phase (including every single α grain) to be elastically softening, so as to facilitate the nucleation of γ from α with a specific crystallographic orientation relationship. This softening-associated phase transition provides a reasonable explanation of the critical temperature T c , as expected from our experimentally determined c ′( T ). Also shown in the inset of Fig. 4 is the 0.2% macroscopic yield strength ( σ y ) determined from the engineering stress–strain curves. Like c ′, σ y exhibits a strong temperature dependency, particularly a considerable yield strength drop above 400 °C, which is consistent with previous studies in the literature [9] , [38] , [39] . As described earlier, the yield strength is essentially determined by the grains whose orientation, relative to the loading axis, favours easy activation of dislocation slip. For this NFA, the <110>//LD grains yield first upon plastic deformation; the microscopic yield strength ( ) with respect to the <110>//LD grains also decreases significantly as the temperature increases, as shown in Table 1 . It is known that the dislocation character determines the onset of crystallographic slip, and the elastic energy factor ( K ) of a dislocation may be considered as a strength indicator [34] , [37] . For example, the energy factor for straight edge dislocations with a Burgers vector of a ‹100› and a dislocation line direction of [001] (denoted here as 100[001]) can be evaluated as (refs 34 , 37 ). The calculated K -values, as listed in Table 1 , appear to scale with the yield strength, although K shall be slightly smaller (<10%) for temperatures below 600 °C where the a /2<111> dislocations (for example, ) dictate the yielding [34] . This behaviour suggests that, in addition to less dispersion strengthening from the NCs and possible grain-boundary-mediated softening (for example, dislocation adsorption, and so on) at increased temperatures [9] , the yield strength drop could be also induced by the reduction of the shear stiffness ( c ′) or, in other words, the large elastic anisotropy. Qualitatively, this finding may be understood in the framework of refs 34 , 37 which showed that dislocation pile-ups can be markedly influenced by c ′ when full anisotropic elasticity is considered. The anisotropy-induced intergranular strains/stresses in the <110>//LD grains at RT, 400 and 600 °C show a nearly identical accumulation process during the onset of yielding and in the subsequent early-stage plastic deformation regime (see the inset of Fig. 5 ). This intriguing similarity indicates that the same yielding mechanism is dominated by dislocation slip inside the grains, as manifested by the unaltered lattice strains and the increased intergranular strains/stresses. However, at high temperatures from 750 to 800 °C, the onset of yielding is immediately followed by lattice softening as seen from decreased lattice strains; this implies that these grains sustain less and less loads, and the plastic deformation is mediated by grain-boundary activities, although the Y-Ti-O NCs and vacancy-solute interactions retard diffusion [40] . It is also noted that, in response to higher values of plastic deformation, a deformation crossover exists from low-temperature strain hardening to high-temperature strain softening; the crossover temperature lies between 400 and 600 °C. This crossover phenomenon demonstrates that intragranular dislocation activities dictate the late-stage of plastic deformation at low temperatures, whereas intergranular grain boundary activities are predominant at high temperatures. It should be noted that the volume fraction of NCs in a 14YWT NFA can be estimated to be <0.1%, in consideration of their sizes of ~1-2 nm diameter with a number density of 1 × 10 23 m −3 (refs 9 , 17 , 41 ). Moreover, these NCs have been characterized to be coherent with the ferrite matrix [5] , [17] . Such a small volume fraction, together with the nanocluster-matrix coherency, would give rise to negligibly small misfit strains and stress concentrations, if any, between NCs and the ferrite matrix during elastic deformation. Thus, NCs are believed to have insignificant effect on the single-crystal elastic constants of the ferrite matrix. This may explain why there is no great difference in elastic constants between NFAs and Fe (or conventional steels), as assumed in many studies [9] . However, there has been no direct measurement of the single-crystal elastic constants of NFAs to prove this hypothesis. In this regard, our diffraction results provide the first experimental evidence for validating this scenario. In summary, anisotropic responses of the ultrafine 14 YWT NFA grains when subjected to tensile stresses at a broad range of temperatures were investigated using in situ neutron diffraction. Temperature-dependent single-crystal elastic constants for the NFA were determined using a new model developed in the present work that takes into account the effect of preferred grain orientations. A strong temperature-dependent elastic anisotropy is revealed as a result of a sharp decrease in the shear stiffness constant, indicating elastic softening and instability of the ferritic matrix at elevated temperatures. The anisotropy-induced intergranular strain/stress accumulations reveal a crossover phenomenon of plastic deformation from a low-T intragranular dislocation slip mechanism to that mediated by grain boundary activities at high-T. This study provides unique insights into the grain-level mesoscale deformation mechanisms. Alloy synthesis The 14YWT NFA was made by mechanical alloying of the mixture of Fe-Cr-W-Ti alloy powder and Y 2 O 3 powder, followed by canning in an evacuated jacket and hot extrusion at 850 °C. The hot-extruded ingot was then annealed for 1 h at 1,000 °C. One heat was used to produce this NFA, whose nominal composition is Fe-14Cr-0.16W-0.4Ti-0.14Y-0.4O (at.%). The details of alloy processing have been described elsewhere [2] . Neutron diffraction experimental setup In situ neutron diffraction experiments were performed on VULCAN [19] , the Engineering Materials Diffractometer at the SNS, Oak Ridge National Laboratory. Threaded dogbone-shaped NFA specimens of 2.90 mm in diameter and 20.6 mm in gauge-length were uniaxially deformed under tension using a Materials Testing System load-frame. The macroscopic engineering strain for the measurement at RT was recorded by an extensometer with a nominal gauge length of 12.7 mm. An induction heater attached to the load-frame was used for heating each specimen to a preset temperature, at which tensile loading of the specimen was conducted while being monitored in situ by neutron diffraction (see Supplementary Fig. 2 ). Four fine-gauge K -type thermocouples were spot weld onto each specimen to control and monitor the temperatures at locations near the specimen centre and the two ends. A uniform temperature zone of ~10 mm in the centre of each specimen was established by fine-tuning the induction heater before loading. This homogeneous zone, having a temperature gradient of <3 °C and being the hottest part of the specimen, was probed in situ by the neutron beam under tensile loading with a strain rate of ~8 × 10 −5 s −1 . True stresses and true strains during plastic deformation at high temperatures were evaluated from measured engineering stresses, together with engineering strains estimated from the relative cross-head displacements after a linear correction (see more details in Supplementary Note 1 ). As shown in Supplementary Fig. 1 , the tensile stress axis of the load-frame was mounted at 45° from the incident neutron beam direction. Diffraction patterns were recorded by the two detector banks (namely, B1 and B2) positioned at diffraction angles of −/+90°. As such, B1 and B2 collected diffraction from the lattice planes perpendicular and parallel to the LD, respectively. The sampling volume was defined by the incident beam slits (5 mm width and 3 mm height) and the radial collimators located between the specimen and the detector banks restricting the field of view to 5 mm along the neutron beam path. The neutron diffraction data were collected continuously during the tensile loading at various temperatures. By using the data reduction software VDRIVE [42] , the recorded data were then ‘sliced’ and binned into histograms corresponding to small temporal intervals that were synchronized with the loading parameters (force, displacement, temperature, and so on.). Single–peak fitting, employing the GSAS program in VDRIVE, was used to extract the peak position, width and intensity corresponding to each hkl reflection. More details about the neutron diffraction experimental setup are available in Supplementary Note 1 . How to cite this article: Stoica, G. M. et al. Temperature-dependent elastic anisotropy and mesoscale deformation in a nanostructured ferritic alloy. Nat. Commun. 5:5178 doi: 10.1038/ncomms6178 (2014).